UNC-43/CaMKII-triggered anterograde signals recruit GABAARs to mediate inhibitory synaptic transmission and plasticity atC. elegansNMJs 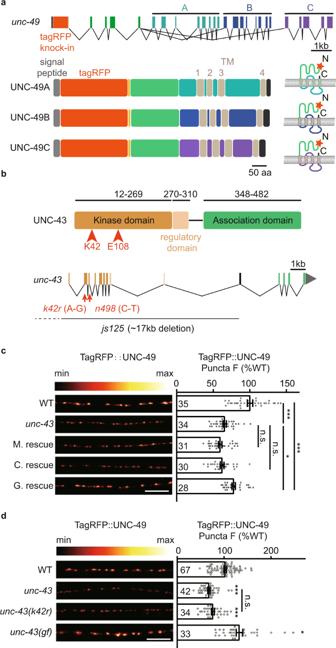Fig. 1: Presynaptic UNC-43/CaMKII regulates postsynaptic GABAAR abundance at GABAergic synapses. aSchematic representation of thexj1024locus. A tagRFP coding sequence was inserted before the first exon shared by UNC-49A, UNC-49B, and UNC-49C. TagRFP consequently labels the UNC-49A, UNC-49B, and UNC-49C proteins.bThe protein structure of UNC-43 is shown on top. Thejs125mutation has a 17 kb deletion (upstream of the promoter to the 10th exon) that deletes most of the coding sequences. The kinase-dead mutantunc-43(k42r)has a point mutation and causes the K42R coding variant. The gain-of-functionunc-43 (gf) (n498, gain of function) mutant has a point mutation that causes single amino acid substitution E108K.cThe puncta fluorescence intensity marked by TagRFP-UNC-49 (underunc-49own promoter) in dorsal nerve cord axons was decreased in theunc-43mutants. This defect was rescued by transgenic expression of UNC-43 in GABAergic motor neurons (G. rescue), but not by UNC-43 expression in cholinergic neurons (C. rescue) or in body-wall muscles (M. rescue). Representative images (left, scale bar 10 μm, Pseudo-color: Red Hot) and mean puncta intensities +/− SEM (right, Ns represent the number of animals tested) are shown. One-way ANOVA with post-hoc Bonferroni’s multiple comparison test. *p< 0.05, ***p< 0.001, n.s. not significant.dGABAAR fluorescence intensity is decreased in theunc-43(k42r) kinase-dead mutants, and increased in theunc-43(gf) (n498, gain of function) mutants. Representative images (left, scale bar 10 μm, Pseudo-color: Red Hot) and mean puncta intensities + /- SEM (right, Ns represent the number of animals tested) are shown. Kruskal–Wallis test with post-hoc Dunn’s test. *p< 0.05, ***p< 0.001, n.s. not significant. Forc,d, source data are provided as a Source Data file. Disturbed inhibitory synaptic transmission has functional impacts on neurodevelopmental and psychiatric disorders. An essential mechanism for modulating inhibitory synaptic transmission is alteration of the postsynaptic abundance of GABA A Rs, which are stabilized by postsynaptic scaffold proteins and recruited by presynaptic signals. However, how GABAergic neurons trigger signals to transsynaptically recruit GABA A Rs remains elusive. Here, we show that UNC-43/CaMKII functions at GABAergic neurons to recruit GABA A Rs and modulate inhibitory synaptic transmission at C. elegans neuromuscular junctions. We demonstrate that UNC-43 promotes presynaptic MADD-4B/Punctin secretion and NRX-1α/Neurexin surface delivery. Together, MADD-4B and NRX-1α recruit postsynaptic NLG-1/Neuroligin and stabilize GABA A Rs. Further, the excitation of GABAergic neurons potentiates the recruitment of NLG-1-stabilized-GABA A Rs, which depends on UNC-43, MADD-4B, and NRX-1. These data all support that UNC-43 triggers MADD-4B and NRX-1α, which act as anterograde signals to recruit postsynaptic GABA A Rs. Thus, our findings elucidate a mechanism for pre- and postsynaptic communication and inhibitory synaptic transmission and plasticity. Fast synaptic inhibition is mediated by neurotransmitter GABA and GABA-activated chloride channels (GABA A Rs). Disturbed inhibitory synaptic transmission has functional impacts on the pathology of neurodevelopmental and psychiatric disorders (including autism spectrum disorders and depression). An essential mechanism for modulating inhibitory synaptic transmission and plasticity is altering the postsynaptic abundance of GABA A Rs [1] . Long-term potentiation and inhibition of GABAergic transmission have been associated with increased or decreased GABA A R synaptic abundance, respectively [2] , [3] . Like other postsynaptic receptors, GABA A Rs at the cell surface undergo lateral diffusion and require postsynaptic scaffolds to stabilize their synaptic enrichment [2] , [3] , [4] , [5] . In mammals, GABA A R clustering and anchoring are mediated by complex inhibitory postsynaptic scaffolds major consist of gephrin, collybistin, Neuroligin-2, and LHFPL4/GARLH4 [5] , [6] , [7] , [8] , [9] , [10] , [11] , [12] , [13] , [14] . Previous research has shown that the GABA A Rs are stabilized by distinct scaffolds at C. elegans neuromuscular junctions (NMJs), including the synaptic adhesion molecule NLG-1/Neuroligin, and the FERM domain-containing protein FRM-3 [15] , [16] , [17] , [18] . The postsynaptic GABA A Rs and inhibitory postsynaptic currents are eliminated in double mutants lacking both NLG-1 and FRM-3 [17] . Besides the postsynaptic scaffolds, the presynaptic neurons also play essential roles in positioning and clustering postsynaptic receptors. During synaptogenesis, the innervation by presynaptic neurons releases anterograde signals to induce receptor aggregation and clustering in the post-junctional membranes. For example, at mammalian cholinergic synapses, cholinergic motor neurons release extracellular proteoglycan agrin to recruit acetylcholine receptors to postsynaptic membranes [19] , [20] , [21] . Other reports have shown that GABAergic motor neurons secrete the ADAMTS-like extracellular protein MADD-4B/Punctin, which promotes the localization of GABA A Rs at inhibitory synapses at NMJs in C. elegans [15] , [16] . In addition, during the induction of activity-dependent synaptic plasticity, the excitation of the presynaptic neurons could trigger the recruitment of postsynaptic receptors and require anterograde signals released by presynaptic neurons. The transsynaptic recruitment of receptors has been extensively studied at excitatory synapses [22] , [23] , [24] , [25] , [26] , [27] . However, how the GABAergic neurons trigger anterograde signals to recruit GABA A Rs remains unclear. Calcium/calmodulin-dependent protein kinase II (CaMKII) is a serine/threonine-specific protein kinase activated by the Ca 2+ /Calmodulin and functions as a ubiquitous mediator of cellular Ca 2+ signals [28] . CaMKII is well known as an essential component of postsynaptic density (PSD) proteins at excitatory synapses [29] , and necessary for NMDA receptor-dependent long-term potentiation (LTP) [30] , [31] , [32] , [33] , [34] , [35] , [36] . At GABAergic synapses, postsynaptic CaMKII has been reported to phosphorylate GABA A Rs within the TM3-4 domain to regulate receptor insertion at the cell surface [37] , [38] , [39] , [40] , [41] . CaMKII is required for the induction of rebound potentiation in Purkinje neurons [42] , [43] , [44] and is also required for the moderate N-methyl-Daspartate receptor (NMDAR)-activating stimuli-induced long-term potentiation of inhibition (iLTP) in hippocampal neurons [2] , [45] . Besides that, it has been known for a long time that CaMKII is expressed and functions on the presynaptic side [35] , [46] , [47] , [48] , [49] , [50] , [51] . However, whether the presynaptic CaMKII could transsynaptically recruit postsynaptic receptors and be involved in inhibitory synaptic transmission and plasticity remain elusive. Here, we utilize the C. elegans NMJs as a model to study how presynaptic neurons trigger anterograde signals to recruit GABA A Rs at inhibitory synapses. We found that UNC-43, the C. elegans ortholog of CaMKII, is required for GABA A Rs recruitment and modulates inhibitory synaptic transmission. Experiments using multiple reporter fusion constructs showed that UNC-43 functions at GABAergic motor neurons to recruit GABA A Rs in the same pathway with NLG-1, but not FRM-3. Next, we demonstrated that UNC-43 promotes presynaptic MADD-4B secretion and cell adhesion molecule NRX-1α/Neurexin GABAergic motor neuron surface delivery. Together, MADD-4B and NRX-1α recruit postsynaptic NLG-1 and stabilize GABA A Rs. Further, we confirmed that the activity-dependent plasticity in the inhibitory synapses requires the presynaptic UNC-43, MADD-4B, and NRX-1α, and is mediated by the NLG-1-stabilized GABA A Rs. Collectively, our work elucidates how presynaptic neurons transsynaptically recruit postsynaptic receptors during synaptogenesis and activity-dependent plasticity. Presynaptic UNC-43/CaMKII regulates postsynaptic GABA A Rs abundance at GABAergic synapses To study the function of CaMKII on inhibitory synaptic transmission, we took advantage of the neuromuscular junction (NMJ) as a synaptic model. In C. elegans , the majority of GABAergic neurons in the nervous system are inhibitory motor neurons that innervate body-wall muscles [52] , [53] , [54] , [55] . At the nerve cord, muscle arms elongate and form synapses with GABAergic axon terminals. As a result, the C. elegans body-wall muscles receive direct synaptic inputs from both cholinergic and GABAergic motor neurons [56] . To visualize endogenous GABA A Rs, we used a similar strategy as the previous report by inserting a tagRFP coding sequence after the signal peptide sequence of the unc-49 gene that encodes GABA A R in C. elegans using the CRISPR-cas9 genome editing system [18] . The tagRFP can label all three GABA A R subunits: UNC-49A, UNC-49B, and UNC-49C (Fig. 1a ). To test whether the tagRFP fused GABA A Rs fold and function well, we performed aldicarb assays to study whether the inhibitory synaptic transmission at NMJs is altered in this tagRFP-tagged GABA A Rs imaging strain; very briefly, the cholinesterase inhibitor aldicarb prevents acetylcholine breakdown, and the attendant acetylcholine accumulation at synapses leads to muscle over-excitation and worm paralysis. Fundamentally, this assay can monitor the alteration of excitatory and inhibitory synaptic transmission [57] . During the 120 minutes of exposure to aldicarb, we found that the paralysis rate of tagRFP knock-in worms did not differ from the wild type (Supplementary Fig. 1 ). In contrast, the unc-49 null mutants showed accelerated paralysis compared to the wild-type worms, thus implying impairment of inhibitory synaptic transmission at NMJs (Supplementary Fig. 1 ) and supporting that our tagRFP-tagged GABA A Rs are functional. Fig. 1: Presynaptic UNC-43/CaMKII regulates postsynaptic GABA A R abundance at GABAergic synapses. a Schematic representation of the xj1024 locus. A tagRFP coding sequence was inserted before the first exon shared by UNC-49A, UNC-49B, and UNC-49C. TagRFP consequently labels the UNC-49A, UNC-49B, and UNC-49C proteins. b The protein structure of UNC-43 is shown on top. The js125 mutation has a 17 kb deletion (upstream of the promoter to the 10th exon) that deletes most of the coding sequences. The kinase-dead mutant unc-43 ( k42r) has a point mutation and causes the K42R coding variant. The gain-of-function unc-43 (gf) (n498 , gain of function) mutant has a point mutation that causes single amino acid substitution E108K. c The puncta fluorescence intensity marked by TagRFP-UNC-49 (under unc-49 own promoter) in dorsal nerve cord axons was decreased in the unc-43 mutants. This defect was rescued by transgenic expression of UNC-43 in GABAergic motor neurons (G. rescue), but not by UNC-43 expression in cholinergic neurons (C. rescue) or in body-wall muscles (M. rescue). Representative images (left, scale bar 10 μm, Pseudo-color: Red Hot) and mean puncta intensities +/− SEM (right, Ns represent the number of animals tested) are shown. One-way ANOVA with post-hoc Bonferroni’s multiple comparison test. * p < 0.05, *** p < 0.001, n.s. not significant. d GABA A R fluorescence intensity is decreased in the unc-43 ( k42r ) kinase-dead mutants, and increased in the unc-43(gf) (n498 , gain of function) mutants. Representative images (left, scale bar 10 μm, Pseudo-color: Red Hot) and mean puncta intensities + /- SEM (right, Ns represent the number of animals tested) are shown. Kruskal–Wallis test with post-hoc Dunn’s test. * p < 0.05, *** p < 0.001, n.s. not significant. For c , d , source data are provided as a Source Data file. Full size image To determine whether UNC-43/CaMKII participates in regulating GABA A R abundance, we used the unc-43(js125) null allele [50] , [58] , which deletes 17 kb of sequence positioned downstream of the promoter and the 10 th exon and lacks most of the sequence encoding UNC-43 (Fig. 1b ). Note that in C. elegans , UNC-43 encodes the sole CaMKII. Quantitative imaging analysis indicated that the GABA A R puncta fluorescence intensity (puncta peak fluorescence to cord fluorescence ratio, peak-to-cord) in the unc-43 mutants was decreased by around 35% compared with wild type (Fig. 1c ), suggesting that UNC-43 does affect GABA A R synaptic abundance. We also examined whether UNC-43 exerts a similar function for cholinergic receptors by measuring the synaptic abundance of two acetylcholine receptors L-AchR (UNC-29) and N-AchR (ACR-16) in the unc-43 mutant animals. However, neither of them presented decreased fluorescent intensities compared to the wild type (Supplementary Fig. 2 ). Together, these findings support that UNC-43 is specifically involved in maintaining GABA A R abundance at inhibitory synapses. UNC-43 is expressed in both pre- and postsynapses at excitatory and inhibitory synapses [35] , [46] , [47] , [48] , [49] , [50] , [51] . At C. elegans NMJs, the excitatory motor neurons innervate and contract muscles, and also synapses onto the inhibitory motor neurons to relax the contralateral muscles to generate the sinusoidal movement [53] . To examine where UNC-43 functions to stabilize the postsynaptic GABA A Rs, we restored UNC-43 expression in GABAergic motor neurons (under the unc-25 promoter), in cholinergic motor neurons (under the unc-17 promoter), or in body-wall muscles (under the myo-3 promoter) (all in the unc-43 mutant background). We found that the decreased synaptic abundance of GABA A Rs in the unc-43 mutant was partially rescued by either UNC-43D or UNC-43G isoform [59] , [60] , [61] in GABAergic motor neurons; no rescue was observed with the cholinergic neuron or body-wall muscle groups (Fig. 1c and Supplementary Fig. 3 ). All of the data supports that UNC-43 functions in the GABAergic motor neurons to stabilize postsynaptic GABA A Rs. Since we observed a partial rescue of GABA A Rs recruitment defects in unc-43 mutants by expressing UNC-43 in the GABAergic motor neurons, therefore, we restored UNC-43 (UNC-43D isoform) expression in pan-neurons (under rab-3 or unc-43 promoter), in both GABAergic and cholinergic motor neurons (under unc-25 promoter+ unc-17 promoter), and in both GABAergic motor neurons and muscle cells (under unc-25 promoter+ myo-3 promoter) in the unc-43 mutants, and we found that the GABA A Rs puncta fluorescence defects in the unc-43 mutants can be fully rescued by expressing UNC-43 in pan-neurons or in both GABAergic and cholinergic motor neurons, but not with both GABAergic motor neurons and muscle cells groups (Supplementary Fig. 3 ). These data suggest that the cholinergic UNC-43 is also involved in GABA A Rs recruitment with unknown mechanisms, and it depends on the GABAergic UNC-43. As a calcium/calmodulin-dependent protein kinase, we next studied whether its kinase activity is required for UNC-43-mediated recruitment of GABA A Rs. We generated a kinase-dead mutant unc-43(k42r) using CRISPR-cas9 and analyzed GABA A R abundance. The GABA A R fluorescence intensity was reduced by about 25% in unc-43(k42r) (Fig. 1d ), indicating that UNC-43’s kinase activity is involved in the recruitment of GABA A Rs. Further, we also analyzed the GABA A R synaptic abundance in the unc-43(n498) gain-of-function allele that bears a constitutively activating mutation E108K in the active site core [62] . The GABA A R fluorescence intensity was significantly increased in the unc-43 mutant (Fig. 1d ), supporting the conclusion that activation of UNC-43 promotes GABA A Rs recruitment. UNC-43/CaMKII is required for the GABAergic synaptic localization of GABA A Rs To further investigate whether the remaining GABA A Rs in the unc-43 mutant are correctly localized at GABAergic synapses, we labeled the GABAergic synapses by fusing the endogenous UNC-57/Endophilin in GABAergic motor neurons with GFP in the tagRFP-tagged GABA A Rs strain using a split GFP complementation system [63] , [64] (Fig. 2a ), and calculated the colocalization coefficient between UNC-57 and GABA A Rs (Fig. 2b ). We found that the colocalization coefficient in the unc-43 mutant was significantly decreased compared with the wild type (0.7770 ± 0.0143 for wild type vs. 0.4848 ± 0.0316 for unc-43 ) (Fig. 2c, d ). Further, GABA A R mislocalization could be rescued by restoring UNC-43 expression in the GABAergic motor neurons (Fig. 2c, d ), indicating that presynaptic UNC-43 is required for the GABAergic synaptic localization of GABA A Rs. Fig. 2: Presynaptic UNC-43/CaMKII is required for the GABAergic synaptic localization of GABA A Rs. a , b Schematic illustration of labeling UNC-57 at the GABAergic motor neurons by split GFP complementary system. Seven copies of the split GFP11 were inserted into the C-terminal of unc-57 genomic loci by CRISPR-Cas9 system. The split GFP1-10 was expressed in GABAergic motor neurons by unc-25 promoters. c , d The colocalization coefficient between GABA A Rs and GABAergic synaptic boutons was decreased in the unc-43 mutants; this was rescued by transgenic expression of UNC-43 in GABAergic motor neurons (G. rescue). Pearson’s correlation coefficients between the intensities of GABAergic bouton marker UNC-57 (green, labeled by UNC-57-split GFP under unc-25 promoter) and postsynaptic GABA A Rs (magenta) were used to assess the localization of GABA A Rs at inhibitory synapses. Representative images ( c -top, scale bar, 10 μm), corresponding line scan curve ( c -bottom), and mean Pearson’s correlation coefficients +/− SEM ( d , Ns represent the number of animals tested) are shown. Kruskal–Wallis test with post-hoc Dunn’s test. *** p < 0.001. Source data are provided as a Source Data file. Full size image Presynaptic UNC-43 modulates inhibitory synaptic transmission at NMJs To determine whether the observed GABA A Rs synaptic recruitment defect in the unc-43 mutants caused impairment of GABAergic synaptic transmission, we patch-clamped body-wall muscles and recorded spontaneous miniature inhibitory postsynaptic currents (mIPSCs). Consistent with the previous report [50] , we observed a dramatic decrease in mIPSC frequency in the unc-43 mutants (Fig. 3a, b ). Besides the mIPSC frequency, the mISPC amplitude was also significantly decreased in the unc-43 mutants (Fig. 3a, c ), implying a defect in postsynaptic GABA A Rs. Further, the decreased mIPSC frequency and amplitude could also be partially recovered by expressing UNC-43 in GABAergic neurons but not by expressing UNC-43 in muscles or cholinergic neurons (Fig. 3a–c ). Fig. 3: Presynaptic UNC-43/CaMKII modulates inhibitory synaptic transmission. a – c Endogenous inhibitory synaptic transmission was assessed by recording mIPSCs from body-wall muscles. The defects of mIPSC in the unc-43 mutants were rescued by transgenic expression of UNC-43 in GABAergic motor neurons (G. rescue), but not by UNC-43 expression in cholinergic neurons (C. rescue) or in body-wall muscles (M. rescue). Representative mIPSC traces ( a ), mIPSC rates ( b , Data are presented as mean values +/− SEM, Ns represent the number of animals tested. ), and the cumulative fraction of mIPSC amplitude ( c ) are shown. Kruskal–Wallis test with post-hoc Dunn’s multiple comparisons. * p < 0.05, ** p < 0.01, *** p < 0.001, n.s. not significant. d Schematic for construction of the unc-43 conditional deletion lines. Two LoxP sites were inserted into the genomic loci (at the promoter and the first intron of UNC-43 K11E8.1a to K11E8.1l) by CRISPR/Cas9, the minigene encoding Cre recombinase under unc-25 and myo-3 promoters were used to knock out unc-43 gene in GABAergic motor neurons (G.cKO) and muscle cells (M.cKO), respectively. e – g Endogenous inhibitory synaptic transmission was assessed by recording mIPSCs from body-wall muscles of unc-43 conditional knockout animals. Representative mIPSC traces ( e ), mIPSC rates ( f , Data are pres e nted as mean values +/− SEM, Ns represent the number of animals tested. ), and the cumulative fraction of mIPSC amplitude ( g ) are shown. Kruskal–Wallis test with post-hoc Dunn’s multiple comparisons. * p < 0.05, *** p < 0.001, n.s. not significant. h , i The GABA-evoked currents in the unc-43 mutants were comparable to that in wild-type animals (WT). Representative responses ( h ) and current amplitude ( i , Data are presented as mean values +/− SEM, Ns represent the number of animals tested.) are shown. Two-tailed and unpaired Student’s t -test. n.s. not significant. For b , c , f , g , i , source data are provided as a Source Data file. Full size image To further confirm UNC-43 functions at GABAergic motor neurons to modulate inhibitory synaptic transmission, we generated worms with a conditional unc-43 deletion in GABAergic motor neurons, or in muscle cells. Briefly, we inserted two LoxP sites at the unc-43 promoter and the first intron, respectively, and drove CRE recombinase expression in the GABAergic motor neurons (under unc-25 promoter) and body-wall muscles (under myo-3 promoter) (Fig. 3d ). We found that unc-43 deletion at the GABAergic motor neurons mimics the phenotype of the unc-43 knockout mutants, showing a significant decrease in mIPSC frequency and amplitude (Fig. 3e–g ). Note that there were no obvious mIPSC frequency or amplitude defects in the strains with unc-43 deletion in the body-wall muscles (Fig. 3e–g ). These results confirm that UNC-43 functions at GABAergic motor neurons to support inhibitory synaptic transmission. To investigate whether the expression and/or surface delivery of GABA A Rs are compromised in the unc-43 mutants, we recorded the 0.2 mM and 0.5 mM GABA-evoked currents, which were unaltered in unc-43 mutants (Fig. 3h–i and Supplementary Fig. 4 ). Thus, the mIPSC amplitude defect in the unc-43 mutants is unlikely to be caused by decreased bulk expression and surface delivery of GABA A Rs. A previous study reported a minor decrease in response to pressure-applied GABA (0.2 mM) in the unc-43 mutant [50] . This discrepancy likely arises from the different protocols of recording. These results verified that UNC-43 is required for both GABA A R synaptic recruitment and inhibitory synaptic transmission. To rule out the possibility that the decreased postsynaptic GABA A Rs in the unc-43 mutant is the secondary result of synaptic structural defects, we measured the puncta fluorescence and intensity of endogenous UNC-57/Endophilin in GABAergic motor neurons in the unc-43 mutant. We observed no significant decrease in puncta fluorescence intensities and densities between wild-type and unc-43 mutants (Supplementary Fig. 5a–c ). Further, we also labeled the endogenous UNC-2/CaV2 in the GABAergic motor neurons with GFP by split GFP complementation system [65] . Both the fluorescence intensity and density of UNC-2-GFP fusion protein were not altered in the unc-43 mutants compared to the wild type (Supplementary Fig. 5d–f ). These results suggested that the GABAergic synapse structure was unaltered. We also ruled out the possibility that the decreased postsynaptic GABA A Rs in the unc-43 mutants result from diminished synaptic GABA transmission or neuropeptide release, as both a previous report and our data have demonstrated that the synaptic abundance of GABA A R was not decreased in the unc-25 mutants (which lack GABA biogenesis), snb-1 mutants, unc-13 mutants (which lack synaptic vesicle release), unc-31 mutants (which lack dense-core vesicle release), and egl-3 (which lack neuropeptide maturation) (Supplementary Fig. 6a–c ) [66] . Further, deletion of unc-43 causes a reduction of GABA A R puncta fluorescence in both snb-1 and unc-25 mutants (Supplementary Fig. 6a–b ), indicating UNC-43 recruits GABA A Rs independent of GABAergic neurotransmission. The increase of GABA A Rs puncta fluorescence in the unc-25 mutants may be caused by synaptic homeostasis. Further, GABA A Rs recruitment is not modulated by the BK channel SLO-1 [50] (Supplementary Fig. 6b ). UNC-43 recruits postsynaptic NLG-1 to stabilize GABA A Rs Our previous work reported that the postsynaptic GABA A Rs are recruited by two distinct scaffolds FRM-3 and NLG-1/neuroligin [15] , [16] , [17] , [18] . To investigate whether UNC-43 functions in a single pathway with FRM-3 or with NLG-1 to stabilize GABA A Rs, we generated unc-43; frm-3 and unc-43; nlg-1 double mutants and then analyzed GABA A R fluorescence intensity at synapses. We observed a further reduction of GABA A R puncta fluorescence intensity in the unc-43; frm-3 double mutants compared to the frm-3 and unc-43 single mutants (Fig. 4a ). However, there was no difference in GABA A R fluorescence intensity between the unc-43; nlg-1 double mutants and the nlg-1 single mutant worms (Fig. 4a ). Besides, Super-resolution microscopy studies by Sora mode showed that the GABA A Rs clustering was significantly decreased in both the unc-43 mutants and the nlg-1 mutants, but not in the frm-3 mutants (Supplementary Fig. 7 ). Further, the increase of GABA A R fluorescence intensity by unc-43(n498) gain-of-function mutation was eliminated in the nlg-1 mutant, but not in the frm-3 mutant (Fig. 4b ), lending more support to the conclusion that UNC-43 functions in a single pathway with NLG-1 to recruit GABA A Rs. Fig. 4: UNC-43/CaMKII acts through a single pathway with NLG-1/neuroligin to recruit GABA A Rs. a The tagRFP-UNC-49 puncta fluorescence intensities in the unc-43 ; nlg-1 double mutants were comparable to the nlg-1 single mutants. Representative images (left, scale bar 10 μm, Pseudo-color: Red Hot) and mean puncta intensities +/− SEM (right, Ns represent the number of animals tested) are shown. Kruskal–Wallis test with two-stage linear step-up procedure of Benjamini, Krieger, and Yekutieli correction for multiple comparisons. * p < 0.05, ** p < 0.01, *** p < 0.001, n.s. not significant. b The tagRFP-UNC-49 puncta fluorescence intensities in the unc-43 (gf) ; nlg-1 double mutants were comparable to the nlg-1 single mutants. Representative images (left, scale bar 10 μm, Pseudo-color: Red Hot) and mean puncta intensities +/− SEM (right, Ns represent the number of animals tested) are shown. One-way ANOVA with two-stage linear step-up procedure of Benjamini, Krieger, and Yekutieli correction for multiple comparisons. *** p < 0.001, n.s. not significant. c UNC-43 does not regulate postsynaptic FRM-3 localization. FRM-3-GFP fluorescence intensities in the body-wall muscles in wild-type and unc-43 mutants were shown. Representative images (left, scale bar 10 μm, Pseudo-color: Fire) and mean puncta intensities +/−  SEM (right, Ns represent the number of animals tested) are shown. Two-tailed and unpaired Student’s t -test. n.s. not significant. d UNC-43 functions in the GABAergic neurons to stabilize postsynaptic NLG-1 localization. NLG-1-GFP fluorescence intensities in the body-wall muscles in wild-type and unc-43 mutants were shown. Representative images (left, scale bar 10 μm, Pseudo-color: Fire) and mean puncta intensities +/−  SEM (right, Ns represent the number of animals tested) are shown. Kruskal–Wallis test with post-hoc Dunn’s test. *** p < 0.001, n.s. not significant. For a – d , source data are provided as a Source Data file. Full size image Next, we tested whether UNC-43 may somehow regulate the postsynaptic localization of NLG-1. We expressed the C-terminal GFP-tagged NLG-1 (under the myo-3 promoter) in the muscle cells of wild-type and unc-43 mutant worms. The GABA A Rs recruitment defects of nlg-1 mutants were rescued by the transgene expression of the C-terminal GFP-tagged NLG-1 in the muscle cells (Supplementary Fig. 8 ). We detected a dramatic decrease in signal intensity for the NLG-1 puncta in the unc-43 mutants (Fig. 4d ). Further, we found that this NLG-1 synaptic abundance defect was rescued by restoring UNC-43 expression in GABAergic motor neurons (Fig. 4d ), indicating presynaptic UNC-43 is required for NLG-1 postsynaptic abundance. It is worth noting that the postsynaptic localization of FRM-3 was unaltered in the unc-43 mutants (Fig. 4c , Supplementary Fig. 8 ). These results suggested the possibility that UNC-43/CaMKII stabilizes synaptic GABA A Rs by recruiting postsynaptic NLG-1. UNC-43 recruits postsynaptic NLG-1 and stabilizes GABA A Rs requiring both NRX-1α and MADD-4B Previous studies have shown that the ADAMTS-like secretion protein MADD-4B/Punctin can be secreted by GABAergic motor neurons, and showed that MADD-4B/Punctin acts partially redundantly with presynaptic NRX-1α/Neurexin to recruit postsynaptic NLG-1 at GABAergic synapses [15] , [16] . Consistent with previous reports, we found that madd-4b and nrx-1 mutations cause an additive defect of NLG-1 synaptic localization (Fig. 5a ); specifically, we detected a further decrease in NLG-1 puncta fluorescence intensity in the madd-4b ; nrx-1 double mutants compared to either of the single mutants (Fig. 5a ). In this context, we test whether UNC-43 may function to recruit NLG-1 in a single pathway with MADD-4B and/or NRX-1α. We analyzed the NLG-1 GABAergic synaptic abundance in the madd-4b ; nrx-1 ; unc-43 triple mutants: the unc-43 deletion did not cause any further reduction in NLG-1 puncta fluorescence intensity as compared to the madd-4b ; nrx-1 double mutants (Fig. 5a ). Together, these results support that a single genetic pathway that includes UNC-43, MADD-4B, and NRX-1α is responsible for the recruitment of postsynaptic NLG-1. Fig. 5: UNC-43/CaMKII’s recruitment of GABA A Rs requires both MADD-4B and NRX-1α. a UNC-43 functions in the same pathway with MADD-4B and NRX-1α to stabilize postsynaptic NLG-1 localization. NLG-1-GFP fluorescence intensities in the body-wall muscles in wild type and mutants were shown. Representative images (left, scale bar 10 μm, Pseudo-color: Fire) and mean puncta intensities +/− SEM (right, Ns represent the number of animals tested) are shown. The data for WT and unc-43 are the same as in Fig. 4c . Kruskal–Wallis test with two-stage linear step-up procedure of Benjamini, Krieger, and Yekutieli correction for multiple comparisons. The scatter plotted data labeled with different letters are significantly different ( p < 0.05). b , c Both MADD-4B and NRX-1α are required for UNC-43’s recruitment of GABA A Rs. TagRFP-UNC-49 fluorescence in dorsal nerve cords in wild type and mutants is shown. Representative images (left, scale bar 10 μm, Pseudo-color: Red Hot) and mean puncta intensities +/− SEM (right, Ns represent the number of animals tested) are shown. In b , Kruskal–Wallis test with two-stage linear step-up procedure of Benjamini, Krieger, and Yekutieli correction for multiple comparisons. The scatter plotted data labeled with different letters are significantly different ( p < 0.05). In c , Kruskal–Wallis test with post-hoc Dunn’s test. ** p < 0.01, *** p < 0.001, n.s. not significant. For a – c , source data are provided as a Source Data file. Full size image We then investigated whether UNC-43’s recruitment of GABA A Rs requires MADD-4B and NRX-1α. Consistent with previous reports [15] , we found that MADD-4B and NRX-1α function redundantly to recruit GABA A Rs: there was a further decrease in the fluorescence intensity of GABA A Rs fusion protein puncta in the madd-4b ; nrx-1 double mutants as compared to both the madd-4b and nrx-1 single mutants (Fig. 5b ). Here we observed a less severe defect of GABA A Rs recruitment in the madd-4b ; and nrx-1 mutants than in previous reports [15] , [16] , it may be caused by different strategies to label GABA A Rs. Note that the deletion of unc-43 further decreases the GABA A R puncta fluorescence intensity in the madd-4b and nrx-1 single mutants (Fig. 5b ), but not in the madd-4b ; nrx-1 double mutants (Fig. 5b ). Further, unc-43(n498) gain-of-function mutation is not able to increase the GABA A R puncta fluorescence intensity in the madd-4b ; nrx-1 double mutants (Fig. 5c ), indicating that UNC-43 recruits postsynaptic GABA A Rs requiring both MADD-4B and NRX-1α. UNC-43 promotes MADD-4B/Punctin secretion and NRX-1α/Neurexin GABAergic motor neuron surface delivery Since UNC-43 requires both MADD-4B and NRX-1α to recruit postsynaptic NLG-1, it is possible that UNC-43 regulates MADD-4 and NRX-1α localization. To study MADD-4B secretion, we expressed a C-terminal GFP-tagged MADD-4B fusion in GABAergic neurons (under the unc-25 promoter), and the MADD-4B-GFP fusion protein is able to rescue the GABA A Rs recruitment defects in the madd-4b mutants (Supplementary Fig. 8 ). A MADD-4B-GFP fluorescent signal was evident in both the nerve cords and coelomocytes. Coelomocytes are scavenger cells that endocytose proteins secreted into the body cavity [67] . Accordingly, the GFP signal in the coelomocytes indicates the secreted MADD-4B, while the fluorescent signal from the dorsal cord indicates the MADD-4B that is retained at the motor neuron axon terminals. Compared to the wild type, there was a significant decrease of MADD-4B-GFP fluorescence intensity in coelomocytes of both the unc-43 knockout and unc-43(k42r) kinase-dead mutants (Fig. 6a, b ), and the MADD-4B signal in both unc-43 mutants dorsal nerve cord was significantly increased (Fig. 6c ). As a result, the decrease of MADD-4B-GFP fluorescence intensity in the coelomocytes and the increase of MADD-4B-GFP fluorescence intensity in the dorsal nerve cord as shown in the unc-43 mutants indicate MADD-4B secretion by GABAergic motor neurons is partially blocked in the unc-43 mutants, thus supporting that UNC-43 promotes MADD-4B secretion and it requires UNC-43’s kinase activity. Fig. 6: UNC-43/CaMKII promotes MADD-4B/Punctin secretion. a Schematic representation of C-terminal GFP-tagged MADD-4B fusion under unc-25 promoter (top) and MADD-4B-GFP expressed in D-type motor neurons, meanwhile the secreted MADD-4B-GFP in body cavity was endocytosed by scavenger cell coelomocytes (bottom). b MADD-4B secretion by GABAergic motor neurons was decreased in the unc-43 knockout and unc-43 (k42r) mutants. Secretion of MADD-4B was measured by analyzing GFP fluorescence intensities in the endolysosomal compartment coelomocytes. Representative images (top, scale bar 5 μm) and mean fluorescence intensities +/− SEM (bottom, Ns represent the number of animals tested) are shown. one-way ANOVA with post-hoc Bonferroni’s multiple comparison test. ** p < 0.01, n.s. not significant. c Puncta fluorescence of MADD-4B-GFP in the dorsal nerve cords was measured in the unc-43 mutants. Representative images (top, scale bar 10 μm, Pseudo-color: Fire) and mean puncta intensities +/− SEM (bottom, Ns represent the number of animals tested) are shown. One-way ANOVA with post-hoc Bonferroni’s multiple comparison test. * p < 0.05, ** p < 0.01, n.s. not significant. For b , c , source data are provided as a Source Data file. Full size image Here we ruled out the possibility that the decreased MADD-4B-GFP fluorescence intensity in coelomocytes in unc-43 mutants is caused by abnormal coelomocyte functions or general defect in presynaptic protein secretion, as the endocytosis of a constitutive GFP secreted from muscle cells or from the GABAergic motor neurons by coelomocytes was not affected by unc-43 mutation (Supplementary Fig. 9 ). To study whether UNC-43 regulates the surface delivery of NRX-1α in GABAergic motor neurons, we expressed a dual-tagged NRX-1α fusion protein by inserting pHluorin at the N-terminus and wrmScarlet at the C-terminus of NRX-1α under the unc-25 promoter (Fig. 7a ). pHluorin is a pH-sensitive version of GFP, and receptors with extracellular domain tagged pHluorin are fluorescent upon insertion in the plasma membrane to expose pHluorin in the extracellular environment (PH > 6). Acidification of the extracellular environment to pH 5.5 quenched all the fluorescence in both wild-type and unc-43 mutants (Supplementary Fig. 10 ), suggesting that all of the fluorescent signals are from the pHluorin-NRX-1 α in the plasma membrane. We observed a dramatic decrease of the pHluorin fluorescent signal in both unc-43 knockout and unc-43 (k42r) mutants (Fig. 7b, c, e ), while the wrmScarlet fluorescence intensities were unaltered (Fig. 7b, d ), indicating that the GABAergic motor neuron surface delivery of NRX-1α, but not its expression or axonal trafficking, was promoted by UNC-43. Fig. 7: UNC-43/CaMKII promotes NRX-1α/neurexin GABAergic motor neuron surface localization. a Schematic representation of N-terminal pH-sensitive GFP pHluorin-tagged and C-terminal wrmScarlet-tagged NRX-1α fusion under unc-25 promoter. pHluorin-NRX-1α are fluorescent upon insertion in the plasma membrane to expose pHluorin in the extracellular environment (pH>6). b – e The surface localization of NRX-1α is decreased in the unc-43 mutants. pHluorin and wrmScarlet dual-labeled NRX-1α was expressed in GABAergic neurons. pHluorin-NRX-1α puncta (green) fluorescence in the dorsal nerve cords was decreased in the unc-43 mutants ( c ). NRX-1α-wrmScarlet puncta (magenta) fluorescence in the dorsal nerve cords was unaltered in the unc-43 mutants ( d ). The averaged fluorescence intensity of pHluorin normalized to wrmScarlet fluorescence intensity in the unc-43 mutants ( e ). Repres e ntative images (top, scale bar 10 μm) and mean puncta intensities +/− SEM (bottom, Ns represent the number of animals tested) are shown. One-way ANOVA with post-hoc Bonferroni’s multiple comparison test for c , d , Kruskal–Wallis test with post-hoc Dunn’s test for e . *** p < 0.001, n.s. not significant. For c – e , source data are provided as a Source Data file. Full size image UNC-43/CaMKII-triggered anterograde signals are required for activity-dependent plasticity at GABAergic synapses Previous research shows that UNC-43 is required for activity-dependent plasticity at PLM-AVA synapses by regulating synaptic AMPARs trafficking after presynaptic neuron excitation or silencing [30] , [33] , [68] , [69] . Thus, we tested whether UNC-43 is also required for activity-dependent plasticity at GABAergic synapses of NMJs. To study the activity-dependent plasticity of GABAergic synapses, we optogenetically activated the GABAergic motor neurons by expressing a channelrhodopsin variant (ChIEF) in the GABAergic motor neurons (under unc-25 promoter) and delivering pulsed blue-light excitation (Fig. 8a ). After 30 min of excitation, we analyzed the GABA A R synaptic abundance and found a significant increase of GABA A R puncta fluorescence intensity compared with controls without all-trans retinal (ATR), and it lasted within 2 h (Fig. 8b, c ). Besides, the colocalization coefficient between the presynaptic marker UNC-57 and GABA A Rs was slightly but significantly increased (Fig. 8d, e ). To study whether the increased GABA A Rs recruitment upon GABAergic motor neuron excitation potentiates inhibitory synaptic transmission, we patch-clamped body-wall muscles and recorded mIPSCs. Both the mIPSCs frequency and amplitude were significantly increased in those animals with GABAergic motor neuron excited compared to controls without all-trans retinal (ATR) (Fig. 8f–h ), supporting that the inhibitory synaptic transmission was also increased. This result indicates the existence of activity-dependent synaptic plasticity at GABAergic synapses. Fig. 8: Induction of activity-dependent plasticity at GABAergic synapses. a Schematic illustration of the blue-light stimulation pattern. b , c The activity-dependent plasticity at GABAergic synapses lasts within two hours. Representative images ( b , scale bar 10 μm, Pseudo-color: Red Hot) and the normalized tagRFP fluorescence intensity before and after GABAergic motor neuron excitation ( c , Data are presented as mean values +/− SEM) are shown. n = 11(ATR(−); −30 min); n = 11(ATR(+); −30 min); n = 28 (ATR(−); 30 min); n = 25 (ATR(+); 30 min); n = 22 (ATR(−); 60 min); n = 24 (ATR(+); 60 min); n = 23 (ATR(−); 120 min); n = 23 (ATR(+); 120 min) animals. Two-tailed and unpaired Student’s t -test. *** p < 0.001, n.s. not significant. d , e The colocalization coefficient between GABA A Rs and GABAergic synaptic boutons was increased after excitation of GABAergic motor neurons; Pearson’s correlation coefficients between the intensities of GABAergic bouton marker UNC-57 (green, labeled by UNC-57-split GFP under unc-25 promoter) and postsynaptic GABA A Rs (magenta) were used to assess the localization of GABA A Rs at inhibitory synapses. Representative images ( d -top, scale bar, 10 μm), corresponding line scan curve ( d -bottom), and mean Pearson’s correlation coefficients +/− SEM ( e , Ns repr e sent the number of animals tested) are shown. Two-tailed and unpaired Student’s t -test. *** p < 0.001. f – h Endogenous inhibitory synaptic transmission was assessed by recording mIPSCs from body-wall muscles in transgenic animals expressing a channelrhodopsin variant (ChIEF) in the GABAergic motor neurons (under unc-25 promoter) after blue-light stimulation with or without all-trans retinal (ATR). Representative mIPSC traces ( f ), mIPSC rates ( g , Data are presented as mean values +/− SEM, Ns represent the number of animals tested. ), and the cumulative fraction of mIPSC amplitude ( h ) are shown. Two-tailed and unpaired Student’s t -test for g and Kolmogorov–Smirnov test for h . ** p < 0.01, *** p < 0.001. For c , e , g , h , source data are provided as a Source Data file. Full size image Next, we studied whether GABAergic activity-dependent plasticity requires UNC-43. We detected no increase of GABA A R puncta fluorescence at synapses afterward in the unc-43 mutant animals, and restoring UNC-43 expression in GABAergic motor neurons rescued the activity-dependent increase of GABA A R recruitment (Fig. 9a ), indicating that the presynaptic UNC-43 is required for the activity-dependent plasticity at GABAergic synapses. Besides, GABAergic activity-dependent plasticity was not eliminated in the unc-43 gain-of-function mutants (Fig. 9a ). Fig. 9: UNC-43/CaMKII is required for activity-dependent plasticity at GABAergic synapses. a Presynaptic UNC-43 is required for activity-dependent GABAergic plasticity. TagRFP-UNC-49 puncta fluorescence intensity was increased after GABAergic motor neuron excitation by ChIEF activation in wild type and in the unc-43 gain-of-function mutants, but not in the unc-43 loss of function mutants, and this was rescued by transgenic expression of UNC-43 in GABAergic motor neurons (G. rescue). Representative images (left, scale bar 10 μm, Pseudo-color: Red Hot) and mean puncta intensities +/− SEM (right, Ns represent the number of animals tested) are shown. Kruskal–Wallis test with two-stage linear step-up procedure of Benjamini, Krieger, and Yekutieli correction for multiple comparisons. * p < 0.05, n.s. not significant. b Schematic illustration of split GFP experimental design to label endogenous UNC-43 at GABAergic motor neurons. Seven copies of the split GFP11 were inserted into the N-terminal of unc-43 genomic loci by the CRISPR-Cas9 system. The split GFP1-10 was expressed in GABAergic motor neurons by unc-25 promoters. c The GABAergic presynaptic localization of UNC-43 was increased after GABAergic motor neuron excitation by ChIEF activation. split GFP labels endogenous UNC-43 in GABAergic neurons. Representative images (left, scale bar 10 μm, Pseudo-color: Fire) and mean puncta intensities +/− SEM (right, Ns represent the number of animals tested) are shown. Two-tailed Mann–Whitney test. 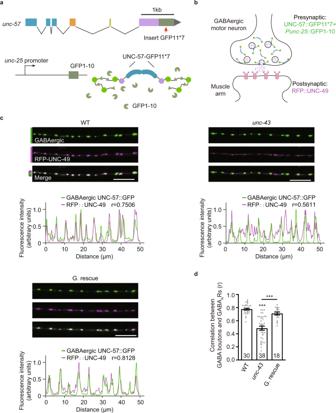Fig. 2: Presynaptic UNC-43/CaMKII is required for the GABAergic synaptic localization of GABAARs. a,bSchematic illustration of labeling UNC-57 at the GABAergic motor neurons by split GFP complementary system. Seven copies of the split GFP11 were inserted into the C-terminal ofunc-57genomic loci by CRISPR-Cas9 system. The split GFP1-10 was expressed in GABAergic motor neurons byunc-25promoters.c,dThe colocalization coefficient between GABAARs and GABAergic synaptic boutons was decreased in theunc-43mutants; this was rescued by transgenic expression of UNC-43 in GABAergic motor neurons (G. rescue). Pearson’s correlation coefficients between the intensities of GABAergic bouton marker UNC-57 (green, labeled by UNC-57-split GFP underunc-25promoter) and postsynaptic GABAARs (magenta) were used to assess the localization of GABAARs at inhibitory synapses. Representative images (c-top, scale bar, 10 μm), corresponding line scan curve (c-bottom), and mean Pearson’s correlation coefficients +/− SEM (d, Ns represent the number of animals tested) are shown. Kruskal–Wallis test with post-hoc Dunn’s test. ***p< 0.001. Source data are provided as a Source Data file. * p < 0.05. d MADD-4B, NRX-1α, and NLG-1, but not FRM-3, are required for activity-dependent plasticity at GABAergic synapses. Representative images (left, scale bar 10 μm, Pseudo-color: Red Hot) and mean puncta intensities +/− SEM (right, Ns represent the number of animals tested) are shown. The data for WT is the same as in a . Kruskal–Wallis test with two-stage linear step-up procedure of Benjamini, Krieger, and Yekutieli correction for multiple comparisons. * p < 0.05, ** p < 0.01, n.s. not significant.For a , c , d , source data are provided as a Source Data file. Full size image Further, we asked whether the presynaptic localization of UNC-43 is altered upon GABAergic motor neuron excitation. To visualize endogenous UNC-43 at GABAergic motor neurons, we utilized the split GFP complementary system [63] , [64] . We used CRISPR/Cas9 system to insert a sequence coding for seven GFP11 fragments at the N-terminus of UNC-43. In parallel, the GFP1-10 fragment was constitutively expressed in the GABAergic motor neurons under the control of the unc-25 promoter (Fig. 9b ) to label the endogenous localization of UNC-43 in GABAergic motor neurons. We observed a significant increase in the GFP fluorescent signal upon blue-light-stimulated GABAergic neuron excitation (Fig. 9c ), supporting the conclusion that more UNC-43 are localized at the GABAergic motor neuron axon terminals upon GABAergic motor neuron stimulation. Since UNC-43 is required for the increase of the synaptic abundance of GABA A Rs after excitation of GABAergic motor neurons, linking with our finding that UNC-43 acts through a single pathway with NLG-1 to recruit GABA A Rs, it is likely that the NLG-1-stabilized diffusing GABA A Rs, rather than the FRM-3-stabilized immobilized GABA A Rs, mediate the inhibitory activity-dependent plasticity. To test this hypothesis, we turned to the nlg-1 and frm-3 mutants. We observed an increase of GABA A Rs recruitment after GABAergic motor neuron excitation in the frm-3 mutants, but not in the nlg-1 mutants (Fig. 9d ), which supports our hypothesis that the diffusing GABA A Rs stabilized by NLG-1 mediate activity-dependent plasticity at inhibitory synapses. To study whether the UNC-43-participated activity-dependent plasticity requires MADD-4B and NRX-1α, we studied the activity-dependent plasticity in the madd-4b; nrx-1 double mutants. Similar to in the unc-43 mutants, the increase of GABA A Rs postsynaptic abundance post GABAergic motor neuron excitation was blocked in the madd-4b ; nrx-1 double mutants (Fig. 9d ). Further, the secretion of MADD-4B and the surface delivery of NRX-1α were both increased upon GABAergic neuron excitation (Supplementary Fig. 11 ), supporting the conclusion that MADD-4 and NRX-1α also participate in the activity-dependent plasticity at GABAergic synapses, and they are very likely to work in the single pathway with UNC-43. In this study, we revealed how UNC-43/CaMKII participates in transsynaptically recruiting GABA A Rs at NMJs. We showed that the presynaptic UNC-43/CaMKII promotes MADD-4B secretion and delivery of the cell adhesion molecule NRX-1α to the surface of GABAergic motor neurons. MADD-4B and NRX-1α act as anterograde signals to recruit postsynaptic NLG-1 and stabilize the GABA A Rs at inhibitory synapses. We further demonstrated that the NLG-1-stabilized GABA A Rs, but not the FRM-3-stabilized GABA A Rs, mediate activity-dependent plasticity at GABAergic synapses, and experimentally confirmed that this mediation requires UNC-43, MADD-4B, and NRX-1α. These mechanistic insights about how presynaptic neurons transsynaptically recruit postsynaptic GABA A Rs deepen our understanding about pre- and postsynaptic communications and inhibitory synaptic plasticity. The presynaptic function of UNC-43/CaMKII Most previous studies of CaMKII have focused on its facilitation of AMPAR recruitment to enhance synaptic strength at postsynapses [30] , [33] . At inhibitory synapses, CaMKII is reported to phosphorylate GABA A Rs and regulates their surface delivery [37] , [38] , [39] , [40] , [41] . 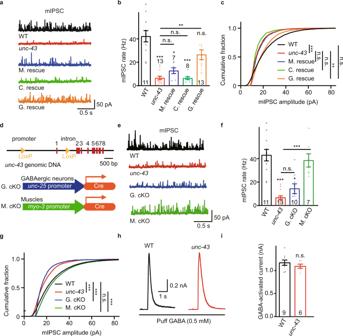Fig. 3: Presynaptic UNC-43/CaMKII modulates inhibitory synaptic transmission. a–cEndogenous inhibitory synaptic transmission was assessed by recording mIPSCs from body-wall muscles. The defects of mIPSC in theunc-43mutants were rescued by transgenic expression of UNC-43 in GABAergic motor neurons (G. rescue), but not by UNC-43 expression in cholinergic neurons (C. rescue) or in body-wall muscles (M. rescue). Representative mIPSC traces (a), mIPSC rates (b, Data are presented as mean values +/− SEM, Ns represent the number of animals tested.), and the cumulative fraction of mIPSC amplitude (c) are shown. Kruskal–Wallis test with post-hoc Dunn’s multiple comparisons. *p< 0.05, **p< 0.01, ***p< 0.001, n.s. not significant.dSchematic for construction of theunc-43conditional deletion lines. Two LoxP sites were inserted into the genomic loci (at the promoter and the first intron of UNC-43 K11E8.1a to K11E8.1l) by CRISPR/Cas9, the minigene encoding Cre recombinase underunc-25andmyo-3promoters were used to knock outunc-43gene in GABAergic motor neurons (G.cKO) and muscle cells (M.cKO), respectively.e–gEndogenous inhibitory synaptic transmission was assessed by recording mIPSCs from body-wall muscles ofunc-43conditional knockout animals. Representative mIPSC traces (e), mIPSC rates (f, Data are presented as mean values +/− SEM, Ns represent the number of animals tested.), and the cumulative fraction of mIPSC amplitude (g) are shown. Kruskal–Wallis test with post-hoc Dunn’s multiple comparisons. *p< 0.05, ***p< 0.001, n.s. not significant.h,iThe GABA-evoked currents in theunc-43mutants were comparable to that in wild-type animals (WT). Representative responses (h) and current amplitude (i, Data are presented as mean values +/− SEM, Ns represent the number of animals tested.) are shown. Two-tailed and unpaired Student’st-test. n.s. not significant. Forb,c,f,g,i, source data are provided as a Source Data file. In hippocampal neurons, the moderate N-methyl-Daspartate receptor (NMDAR)-activating stimuli cause CaMKII selectively translocating to inhibitory synapses to phosphorylate GABA A R β3S383 and recruit scaffold protein gephyrin, which promotes GABA A Rs accumulation and immobilization at synapses [2] , [45] , [70] . Besides, an acute increase in neuronal activity of cultured hippocampal neurons also promotes the phosphorylation of β3S383 by CaMKII [39] . Further, in cerebellar somatodendritic basket cell synapses, CaMKII is required for the rebound potentiation (RP) by phosphorylation of GABA A Rs receptor [44] . However, many studies have indicated that CaMKII has functional impacts at presynapses [35] , [46] , [47] , [48] , [49] , [50] , [51] . CaMKII is enriched at presynaptic sites, and accounts for ~2% of the total synaptic vesicle protein amount [71] . Presynaptic injection of the membrane-impermeable CaMKII inhibitor peptide 281-309 was shown to block excitatory synaptic plasticity in cultured hippocampal neurons [47] and presynaptic CaMKII was implicated in synaptogenesis and synaptic transmission at NMJs of both Drosophila and C. elegans [46] , [50] . In the present study, we identified a transsynaptic GABA A R recruitment function of presynaptic CaMKII, thus demonstrating CaMKII’s involvement in inhibitory synaptic transmission. We also show that this transsynaptic recruitment activity is supported by MADD-4B secretion and NRX-1α surface delivery and propose the hypothesis that UNC-43-triggered anterograde signals are required for the activity-dependent plasticity at inhibitory synapses. Thus, the function of CaMKII in recruiting postsynaptic GABA A Rs is conserved in species, and both presynaptic and postsynaptic CaMKII can recruit postsynaptic GABA A Rs. Recall our finding that the extent of the synaptic GABA A R abundance defects, MADD-4B secretion defect, and NRX-1α motor neuron surface delivery were similar in the unc-43 null mutant as in worms expressing a kinase-dead mutant unc-43 (k42r) (Fig. 1d , Figs. 6 and 7 ). This suggests that UNC-43’s kinase activity is required to promote MADD-4B secretion and NRX-1α surface delivery to support transsynaptic recruitment of GABA A Rs. NLG-1- and FRM-3-stabilized GABA A Rs Previous studies have demonstrated that GABA A Rs are stabilized by distinct synaptic scaffolds at C. elegans NMJs: there are NLG-1-stabilized GABA A Rs and FRM-3-stabilized GABA A Rs [15] , [16] , [17] , [18] . It has been shown that the NLG-1-stabilized GABA A Rs and FRM-3-stabilized GABA A Rs together mediate inhibitory synaptic transmission [15] , [16] , [17] , [18] . However, it remains unclear which type of receptors mediate inhibitory synaptic plasticity. Here, by using the nlg-1 and frm-3 mutants, we demonstrate that NLG-1-stabilized GABA A Rs mediate activity-dependent plasticity at inhibitory synapses. Further, our study indicates a plausible explanation for how NLG-1-stabilized GABA A Rs are recruited to inhibitory postsynaptic elements upon excitation of presynaptic GABAergic motor neurons: it is likely that Ca 2+ influx after GABAergic motor neuron excitation activates UNC-43, which can trigger more MADD-4B secretion and NRX-1α surface delivery. These molecules can subsequently act as anterograde signals to recruit additional NLG-1 to postsynaptic elements to somehow help stabilize the GABA A Rs. Given that no physical interactions have yet been reported between NLG-1 and GABA A Rs, the nature of this stabilization remains unclear. A recent study proposed that FRM-3 and CASK ortholog LIN-2 mediate the interaction between NLG-1 and GABA A Rs [18] . However, an additive defect in GABA A Rs recruitment and inhibitory synaptic transmission was observed in the frm-3; nlg-1 double mutant [17] . Further, UNC-43 functions in a single pathway with NLG-1 to recruit GABA A Rs, but not with FRM-3. In summary, the current data does not support the conclusion that NLG-1 recruits GABA A Rs through FRM-3. Contact for reagent and resource sharing Further information and requests for resources and reagents should be directed to and fulfilled by the Lead Contact Xia-Jing Tong (tongxj@shanghaitech.edu.cn). Animals All C. elegans strains were derived from the wild-type Bristol N2 (Caenorhabditis Genetics Center) strain. Worms were cultivated at 20 °C on nematode growth medium (NGM) plates seeded with Escherichia coli ( E. coli ) under standard conditions. The OP50 strain of E. coli was used as a food source for all experiments, except where the HB101 strain was utilized for the electrophysiology study. The well-fed young-adult hermaphrodites were used in all experiments except for coelomocyte imaging experiment in which the adult day-5 animals were used. Transgenic animals were prepared by microinjection, and integrated transgenes were isolated following UV irradiation or by single-copy insertion mediated by miniMos or CRISPR-cas9. A complete list of the strains used in this study can be found in Supplementary data 1 . Molecular information on unc-43 mutants. The js125 mutation is a deletion from 10 kb upstream of the transcription initiation site to exon 10 [50] , [58] . The kinase-dead mutant unc-43(k42r) was generated by CRISPR-cas9, which caused the K42R coding variant. The gain-of-function unc-43 (n498) mutation is a point mutation that causes single amino acid substitution (E108K) and makes the kinase partially active even in the absence of Ca 2+ . Molecular information on madd-4B mutants. The xj0739 mutation is a C insertion in the first exon of madd-4B , introducing an early stop codon and generating a 21 amino acids (aa) product. Plasmids The constructs used and created in this study are detailed in Supplementary data 2 . Primers The primers used in this study are detailed in Supplementary data 3 . Reagents, software, and algorithms The reagents, software, and algorithms used in this study are detailed in Supplementary data 4 . Genome editing by CRISPR-cas9 The tagRFP-T-unc-49(xj1024) knock-in was generated based on the CRISPR-cas9 technique previously described [72] . The tagRFP-T with 3x GS linker was inserted between Gln23 and Asp24, and an extra Gln was added before Asp24 to guarantee the UNC-49 signal peptide coding sequence integrity. The sgRNAs were designed on CRISPR ( http://crispor.tefor.net/ ) [73] . The single-stranded repair template was generated by overlap extension PCR (purified and heated at 95 °C for 5 min). To remove off-target mutations, the transgenic worms were outcrossed with N2 and used for further studies. Similarly, the unc-43(k42r) allele was also generated by CRISPR-cas9. A 99 bp single-stranded repair template was synthesized and purified before injection. The unc-43(xj764[LoxP::unc-43p::unc-43::LoxP]) allele was generated for unc-43 conditional knockout. The first LoxP with EcoRI restriction enzyme cutting site was inserted upstream of unc-43 promoter (3 kb before exon 1 of UNC-43 transcripts K11E8.1a to K11E8.1 l ), and the second LoxP with EcoRI was inserted into the first intron. Under the action of Cre recombinase driven by the tissue-specific promoter, about 3800 bp genomic DNA containing the promoter and 59 bp coding sequence of UNC-43 transcripts (K11E8.1a to K11E8.1l) including start codon was tissue-specifically removed. For the transcript K11E8.1r, the deletion of the 59 bp coding sequence causes a frameshift and an early stop codon. myo-3 and unc-25 promoters were cloned into pFX_NLS::Cre vector [74] . The conditional knockout animals were verified by PCR and sequencing. The unc-57::GFP11*7(xj1544) and GFP11*7-unc-43(xj1455) allele was generated for tissue-specific labeling UNC-57 and UNC-43. unc-57::GFP11*7(xj1544) , seven copies of the GFP11 coding sequence were inserted at the C-terminus of the unc-57 genomic locus. Briefly, GGGS (linker)-GFP11*7 coding sequence was inserted before the stop codon of unc-57 isoforms (T04D1.3a to T04D1.3d). For GFP11*7-unc-43(xj1455) , seven copies of the GFP11 coding sequence were inserted at the N-terminus of the unc-43 genomic locus. Briefly, GGGS (linker)-GFP11*7-GGGS (linker) coding sequence was inserted after the start codon of unc-43 isoforms (K11E8.1b to K11E8.1l). In parallel, the GFP 1-10 fragment was constitutively expressed in the GABAergic motor neurons. As a result, the endogenous UNC-57 and UNC-43 localized in the GABAergic neurons can be visualized. Generation of single-copy insertion alleles by miniMos N2 worms were injected with 10 ng/μL of PCFJ910 plasmid-of-interest containing the promoter and open reading frame (contains a Neomycin resistance gene), 50 ng/μL of pCFJ601 (Mos1 transposase), 10 ng/μL of pGH8 (Prab-3::mCherry), 2.5 ng/μL of pCFJ90 (Pmyo-2::mCherry), and 5 ng/μL of pCFJ104 (Pmyo-3::mCherry). Animals were grown under 25 °C after injection. Neomycin (G418) was added to plates 24 h after injection at a final concentration of 1.5 μg/μL. Homozygous animals with the desired insertion were verified by PCR and sequencing. The xjSi0009 allele encodes GFP-tagged MADD-4B driven by GABAergic motor neuron-specific unc-25 promoter. The GFP sequence was inserted after Phe711 of the MADD-4B coding sequence. The xjSi0016 allele encodes dual-tagged NRX-1α driven by the unc-25 promoter. The pHluorin sequence was inserted between Ile29 and Ile30 of NRX-1α, and the wrmScarlet was inserted after Val1540. Microscopy For UNC-49, UNC-29, UNC-57, UNC-43, FRM-3, and NLG-1 puncta fluorescence imaging, images were captured using a 100x objective (NA = 1.4) on an Olympus microscope (BX53). For ACR-16, MADD-4B, and NRX-1α puncta fluorescence imaging, images were captured using a Nikon 60×1.4 NA objective on a Nikon spinning-disk confocal system (Yokogawa CSU-W1). Young-adult worms were immobilized with 30 μg/μl 2,3-Butanedione monoxime (Sigma). The maximum intensity of dorsal cord projections of Z-series stacks was obtained by Metamorph software (Molecular Devices). Line scans were analyzed in Igor Pro (WaveMetrics) using a custom script [75] . The mean fluorescence intensities of reference FluoSphere microspheres (0.5 μm, ThermoFisher Scientific) were measured during each experiment that controlled for changes in illumination intensities. Automatic image analysis was performed as in previous reports [76] . Briefly, four image parameters were defined: (1) Peak (F peak ): Absolute peak fluorescence, is the averaged ratio of peak fluorescence to the bead standard of the cord analyzed; (2) Cord (F cord ): absolute axon fluorescence, which is the ratio of baseline fluorescence to the bead standard; (3) Puncta F: peak-to-cord magnitude, 100X (F peak – F cord )/F cord ; (4) Density: is the number of peaks found per 10 μm of cord analyzed. All fluorescence values are normalized to wild-type controls to facilitate comparison. To assess the synaptic accumulation of fluorescent proteins, we used the Puncta F: peak-to-cord magnitude. For colocalization assay, images were captured using a 100x objective (NA = 1.4) on an Olympus microscope (BX53). The maximum intensity of dorsal cord projections of Z-series stacks was obtained by ImageJ. The background was removed using the Subtract Background plugin of Image J (rolling ball radius 50 pixels). The fluorescence intensity along the cord was evaluated with the Plot Profile plugin (line width 20 pixels). For each channel, the values were normalized to the value of maximal intensity. To assess the correlations between GABAergic boutons and GABA A Rs, the mean of Pearson’s coefficients between the distribution of fluorescence intensity in each channel were compared in Figs. 2d and 8e . For coelomocytes imaging, images were captured using a Nikon 60 × 1.4 NA objective on a Nikon spinning-disk confocal system (Yokogawa CSU-W1). 5-day adult worms were immobilized with 30 μg/μl 2,3-Butanedione monoxime. All fluorescence values are normalized to wild-type controls to facilitate comparison. To assess fluorescence intensities of coelomocytes, region of interests (ROIs) were traced for the coelomocytes and a background area outside of the animal in ImageJ. Maximum intensities of these ROIs were exported, and fluorescence intensity was corrected for background intensity. Super-resolution microscopy Super-resolution images were captured with a Nikon 60 × 1.4 NA Objective on a Nikon spinning-disk confocal system (Yokogawa CSU-W1 SoRa) based on SoRa mode. Live young adult animals were anesthetized with 30 μg/μl 2,3-Butanedione monoxime (Sigma) and the regions of dorsal cords were excited by a 561 nm laser (50% power, 400 ms exposure time). The maximum intensity of dorsal cord projections of Z-series stacks was obtained by ImageJ. The number of animals with diffusing or punctate GABA A Rs was assessed and analyzed by Chi-square test. Aldicarb assay The aldicarb assay was performed as previously described [77] . Briefly, 1 mM aldicarb was added to the NGM plate. More than 20 animals at the young-adult stage were picked on each plate. The paralyzed animals were counted every 10 min. At least three double-blind replicates were performed for each genotype. Electrophysiology Electrophysiology was conducted on dissected C. elegans as previously described [17] . Worms were superfused in the extracellular solution (127 mM NaCl, 5 mM KCl, 26 mM NaHCO 3 , 1.25 mM NaH 2 PO 4 , 20 mM glucose, 1 mM CaCl 2 , and 4 mM MgCl 2 , bubbled with 5% CO 2 , 95% O 2 ) at 22 °C. Whole-cell recordings were carried out with the internal solution (105 mM CH 3 O 3 SCs, 10 mM CsCl, 15 mM CsF, 4 mM MgCl 2 , 5 mM EGTA, 0.25 mM CaCl 2 , 10 mM HEPES, and 4 mM Na 2 ATP). The solution was adjusted to pH 7.2 using CsOH) at 0 mV for mIPSCs. For GABA-activated current recordings, 0.2 or 0.5 mM GABA was pressure ejected for 1.0 s onto body muscles of adult worms. Activity-dependent plasticity assay To prepare the standard agar plates for optogenetic activation of GABAergic motor neurons, 1.6 mM of all-trans retinal (ATR, 100 mM dissolved in ethanol) or ethanol (control) was mixed with OP50 E. coli culture and spotted on 3.5 mm NGM plates. Plates were allowed to dry for 24 h before use. L4 transgenic worms with channelrhodopsin variant CHIEF expressed in the GABAergic motor neurons were transferred to ATR plates and grown overnight. Young adult worms were received pulsed blue-light excitation (460 nm wavelength, 2.4 mW/mm 2 power) at 20 Hz for 30 min, and subjected to GABA A Rs puncta fluorescence analysis or electrophysiology. Statistical analysis All data were presented as mean ± SEM (standard error of the mean) with a scatter plot. Data were analyzed with Prism 8.0 (v8.0.2, GraphPad Software, Inc.). The Kolmogorov–Smirnov test was performed to determine whether the data were normally distributed. For comparison of the two groups, a two-tailed unpaired Student’s t -test (for the normally distributed data, Figs. 3 i, 4 c, 8 c, e, g and Supplementary Figs. 2 b, d, 4 , 5 c, e, f ,) or a two-tailed Mann–Whitney test (for the non-normal data, Fig. 9c and Supplementary Fig. 5 b, 9 a–b, 11a–b ) was performed. For the comparison of more than two and less than six groups, one-way ANOVA with post-hoc Bonferroni’s multiple comparison test (for the normally distributed data, Figs. 1 c, 6 b, c, 7c, d and Supplementary Fig. 6c ) or Kruskal–Wallis test with post-hoc Dunn’s test (for the non-normal data, Figs. 1 d, 2 d, 3 b, f, 4 d, 5 c, 7e and Supplementary Fig. 6a ) or was performed. For the comparison of more than six groups, one-way ANOVA with two-stage linear step-up procedure of Benjamini, Krieger, and Yekutieli correction for multiple comparisons (for the normally distributed data, Fig. 4b and Supplementary Figs. 3 , 6 b, 8 ) or Kruskal–Wallis test with two-stage linear step-up procedure of Benjamini, Krieger, and Yekutieli correction for multiple comparisons (for the non-normal data, Figs. 4 a, 5 a, b, 9 a, d ) was performed. For the comparison of cumulative fractions, a Kolmogorov–Smirnov test (two group, Fig. 8h ) or a Kruskal–Wallis tests with post-hoc Dunn’s test (more than two group, Figs. 3 c, g ) were performed. For Supplementary Fig. 7b , Chi-square tests were performed. 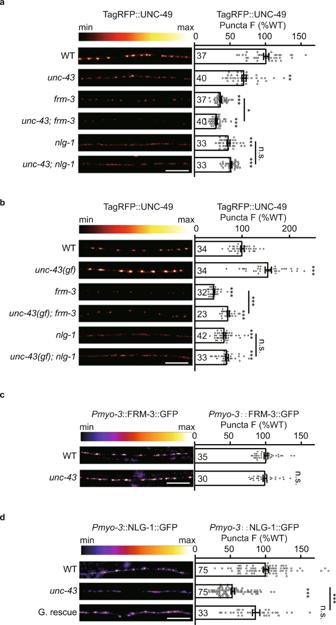Fig. 4: UNC-43/CaMKII acts through a single pathway with NLG-1/neuroligin to recruit GABAARs. aThe tagRFP-UNC-49 puncta fluorescence intensities in theunc-43;nlg-1double mutants were comparable to thenlg-1single mutants. Representative images (left, scale bar 10 μm, Pseudo-color: Red Hot) and mean puncta intensities +/− SEM (right, Ns represent the number of animals tested) are shown. Kruskal–Wallis test with two-stage linear step-up procedure of Benjamini, Krieger, and Yekutieli correction for multiple comparisons. *p< 0.05, **p< 0.01, ***p< 0.001, n.s. not significant.bThe tagRFP-UNC-49 puncta fluorescence intensities in theunc-43 (gf);nlg-1double mutants were comparable to thenlg-1single mutants. Representative images (left, scale bar 10 μm, Pseudo-color: Red Hot) and mean puncta intensities +/− SEM (right, Ns represent the number of animals tested) are shown. One-way ANOVA with two-stage linear step-up procedure of Benjamini, Krieger, and Yekutieli correction for multiple comparisons. ***p< 0.001, n.s. not significant.cUNC-43 does not regulate postsynaptic FRM-3 localization. FRM-3-GFP fluorescence intensities in the body-wall muscles in wild-type andunc-43mutants were shown. Representative images (left, scale bar 10 μm, Pseudo-color: Fire) and mean puncta intensities +/−  SEM (right, Ns represent the number of animals tested) are shown. Two-tailed and unpaired Student’st-test. n.s. not significant.dUNC-43 functions in the GABAergic neurons to stabilize postsynaptic NLG-1 localization. NLG-1-GFP fluorescence intensities in the body-wall muscles in wild-type andunc-43mutants were shown. Representative images (left, scale bar 10 μm, Pseudo-color: Fire) and mean puncta intensities +/−  SEM (right, Ns represent the number of animals tested) are shown. Kruskal–Wallis test with post-hoc Dunn’s test. ***p< 0.001, n.s. not significant. Fora–d, source data are provided as a Source Data file. For the comparison of curves, two-way ANOVA was performed (Supplementary Fig. 1 ). P -value in all figures is donated as n.s. >0.05, * <0.05, ** <0.005, *** <0.001 (expect Fig. 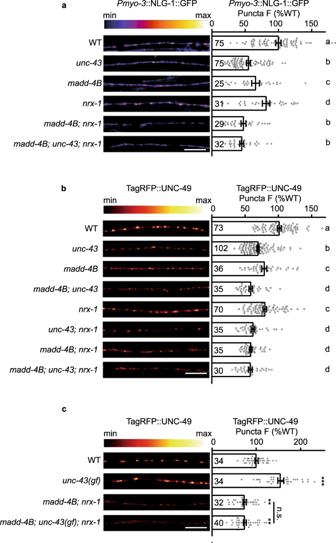Fig. 5: UNC-43/CaMKII’s recruitment of GABAARs requires both MADD-4B and NRX-1α. aUNC-43 functions in the same pathway with MADD-4B and NRX-1α to stabilize postsynaptic NLG-1 localization. NLG-1-GFP fluorescence intensities in the body-wall muscles in wild type and mutants were shown. Representative images (left, scale bar 10 μm, Pseudo-color: Fire) and mean puncta intensities +/− SEM (right, Ns represent the number of animals tested) are shown. The data for WT andunc-43are the same as in Fig.4c. Kruskal–Wallis test with two-stage linear step-up procedure of Benjamini, Krieger, and Yekutieli correction for multiple comparisons. The scatter plotted data labeled with different letters are significantly different (p< 0.05).b,cBoth MADD-4B and NRX-1α are required for UNC-43’s recruitment of GABAARs. TagRFP-UNC-49 fluorescence in dorsal nerve cords in wild type and mutants is shown. Representative images (left, scale bar 10 μm, Pseudo-color: Red Hot) and mean puncta intensities +/− SEM (right, Ns represent the number of animals tested) are shown. Inb, Kruskal–Wallis test with two-stage linear step-up procedure of Benjamini, Krieger, and Yekutieli correction for multiple comparisons. The scatter plotted data labeled with different letters are significantly different (p< 0.05). Inc, Kruskal–Wallis test with post-hoc Dunn’s test. **p< 0.01, ***p< 0.001, n.s. not significant. Fora–c, source data are provided as a Source Data file. 5a, b and Supplementary Fig. 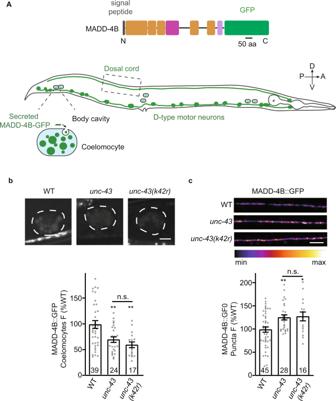Fig. 6: UNC-43/CaMKII promotes MADD-4B/Punctin secretion. aSchematic representation of C-terminal GFP-tagged MADD-4B fusion underunc-25promoter (top) and MADD-4B-GFP expressed in D-type motor neurons, meanwhile the secreted MADD-4B-GFP in body cavity was endocytosed by scavenger cell coelomocytes (bottom).bMADD-4B secretion by GABAergic motor neurons was decreased in theunc-43knockout andunc-43 (k42r)mutants. Secretion of MADD-4B was measured by analyzing GFP fluorescence intensities in the endolysosomal compartment coelomocytes. Representative images (top, scale bar 5 μm) and mean fluorescence intensities +/− SEM (bottom, Ns represent the number of animals tested) are shown. one-way ANOVA with post-hoc Bonferroni’s multiple comparison test. **p< 0.01, n.s. not significant.cPuncta fluorescence of MADD-4B-GFP in the dorsal nerve cords was measured in theunc-43mutants. Representative images (top, scale bar 10 μm, Pseudo-color: Fire) and mean puncta intensities +/− SEM (bottom, Ns represent the number of animals tested) are shown. One-way ANOVA with post-hoc Bonferroni’s multiple comparison test. *p< 0.05, **p< 0.01, n.s. not significant. Forb,c, source data are provided as a Source Data file. 3 , which marked with letters and data corresponding to scatter plots labeled with different letters are significantly different). 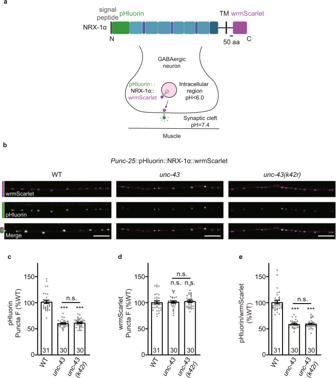Fig. 7: UNC-43/CaMKII promotes NRX-1α/neurexin GABAergic motor neuron surface localization. aSchematic representation of N-terminal pH-sensitive GFP pHluorin-tagged and C-terminal wrmScarlet-tagged NRX-1α fusion underunc-25promoter. pHluorin-NRX-1α are fluorescent upon insertion in the plasma membrane to expose pHluorin in the extracellular environment (pH>6).b–eThe surface localization of NRX-1α is decreased in theunc-43mutants. pHluorin and wrmScarlet dual-labeled NRX-1α was expressed in GABAergic neurons. pHluorin-NRX-1α puncta (green) fluorescence in the dorsal nerve cords was decreased in theunc-43mutants (c). NRX-1α-wrmScarlet puncta (magenta) fluorescence in the dorsal nerve cords was unaltered in theunc-43mutants (d). The averaged fluorescence intensity of pHluorin normalized to wrmScarlet fluorescence intensity in theunc-43mutants (e). Representative images (top, scale bar 10 μm) and mean puncta intensities +/− SEM (bottom, Ns represent the number of animals tested) are shown. One-way ANOVA with post-hoc Bonferroni’s multiple comparison test forc,d, Kruskal–Wallis test with post-hoc Dunn’s test fore. ***p< 0.001, n.s. not significant. Forc–e, source data are provided as a Source Data file. 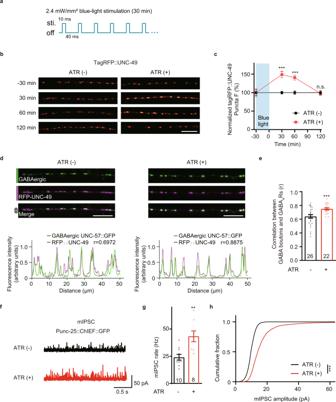Fig. 8: Induction of activity-dependent plasticity at GABAergic synapses. aSchematic illustration of the blue-light stimulation pattern.b,cThe activity-dependent plasticity at GABAergic synapses lasts within two hours. Representative images (b, scale bar 10 μm, Pseudo-color: Red Hot) and the normalized tagRFP fluorescence intensity before and after GABAergic motor neuron excitation (c, Data are presented as mean values +/− SEM) are shown.n= 11(ATR(−); −30 min);n= 11(ATR(+); −30 min);n= 28 (ATR(−); 30 min);n= 25 (ATR(+); 30 min);n= 22 (ATR(−); 60 min);n= 24 (ATR(+); 60 min);n= 23 (ATR(−); 120 min);n= 23 (ATR(+); 120 min) animals. Two-tailed and unpaired Student’st-test. ***p< 0.001, n.s. not significant.d,eThe colocalization coefficient between GABAARs and GABAergic synaptic boutons was increased after excitation of GABAergic motor neurons; Pearson’s correlation coefficients between the intensities of GABAergic bouton marker UNC-57 (green, labeled by UNC-57-split GFP underunc-25promoter) and postsynaptic GABAARs (magenta) were used to assess the localization of GABAARs at inhibitory synapses. Representative images (d-top, scale bar, 10 μm), corresponding line scan curve (d-bottom), and mean Pearson’s correlation coefficients +/− SEM (e, Ns represent the number of animals tested) are shown. Two-tailed and unpaired Student’st-test. ***p< 0.001.f–hEndogenous inhibitory synaptic transmission was assessed by recording mIPSCs from body-wall muscles in transgenic animals expressing a channelrhodopsin variant (ChIEF) in the GABAergic motor neurons (underunc-25promoter) after blue-light stimulation with or without all-trans retinal (ATR). Representative mIPSC traces (f), mIPSC rates (g, Data are presented as mean values +/− SEM, Ns represent the number of animals tested.), and the cumulative fraction of mIPSC amplitude (h) are shown. Two-tailed and unpaired Student’st-test forgand Kolmogorov–Smirnov test forh. **p< 0.01, ***p< 0.001. Forc,e,g,h, source data are provided as a Source Data file. 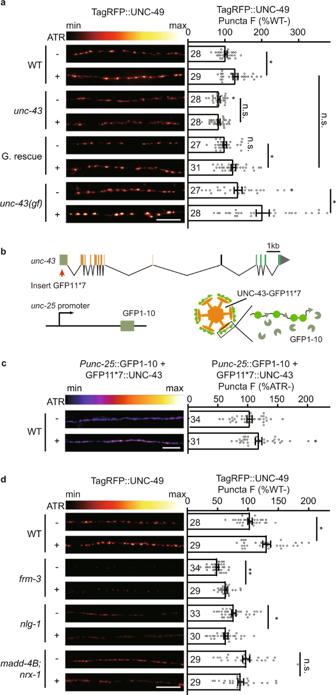Fig. 9: UNC-43/CaMKII is required for activity-dependent plasticity at GABAergic synapses. aPresynaptic UNC-43 is required for activity-dependent GABAergic plasticity. TagRFP-UNC-49 puncta fluorescence intensity was increased after GABAergic motor neuron excitation by ChIEF activation in wild type and in theunc-43gain-of-function mutants, but not in theunc-43loss of function mutants, and this was rescued by transgenic expression of UNC-43 in GABAergic motor neurons (G. rescue). Representative images (left, scale bar 10 μm, Pseudo-color: Red Hot) and mean puncta intensities +/− SEM (right, Ns represent the number of animals tested) are shown. Kruskal–Wallis test with two-stage linear step-up procedure of Benjamini, Krieger, and Yekutieli correction for multiple comparisons. *p< 0.05, n.s. not significant.bSchematic illustration of split GFP experimental design to label endogenous UNC-43 at GABAergic motor neurons. Seven copies of the split GFP11 were inserted into the N-terminal ofunc-43genomic loci by the CRISPR-Cas9 system. The split GFP1-10 was expressed in GABAergic motor neurons byunc-25promoters.cThe GABAergic presynaptic localization of UNC-43 was increased after GABAergic motor neuron excitation by ChIEF activation. split GFP labels endogenous UNC-43 in GABAergic neurons. Representative images (left, scale bar 10 μm, Pseudo-color: Fire) and mean puncta intensities +/− SEM (right, Ns represent the number of animals tested) are shown. Two-tailed Mann–Whitney test. *p< 0.05.dMADD-4B, NRX-1α, and NLG-1, but not FRM-3, are required for activity-dependent plasticity at GABAergic synapses. Representative images (left, scale bar 10 μm, Pseudo-color: Red Hot) and mean puncta intensities +/− SEM (right, Ns represent the number of animals tested) are shown. The data for WT is the same as ina. Kruskal–Wallis test with two-stage linear step-up procedure of Benjamini, Krieger, and Yekutieli correction for multiple comparisons. *p< 0.05, **p< 0.01, n.s. not significant.Fora,c,d, source data are provided as a Source Data file. Reporting summary Further information on research design is available in the Nature Portfolio Reporting Summary linked to this article.